Ballistic to diffusive crossover of heat flow in graphene ribbons Heat flow in nanomaterials is an important area of study, with both fundamental and technological implications. However, little is known about heat flow in two-dimensional devices or interconnects with dimensions comparable to the phonon mean free path. Here we find that short, quarter-micron graphene samples reach ~35% of the ballistic thermal conductance limit up to room temperature, enabled by the relatively large phonon mean free path (~100 nm) in substrate-supported graphene. In contrast, patterning similar samples into nanoribbons leads to a diffusive heat-flow regime that is controlled by ribbon width and edge disorder. In the edge-controlled regime, the graphene nanoribbon thermal conductivity scales with width approximately as ~ W 1.8 0.3 , being about 100 W m −1 K −1 in 65-nm-wide graphene nanoribbons, at room temperature. These results show how manipulation oftwo-dimensional device dimensions and edges can be used to achieve full control of their heat-carrying properties, approaching fundamentally limited upper or lower bounds. The thermal properties of graphene are derived from those of graphite and are similarly anisotropic. The in-plane thermal conductivity of isolated graphene is high, >2,000 W m −1 K −1 at room temperature, due to the strong sp 2 bonding and relatively small mass of carbon atoms [1] , [2] , [3] . Heat flow in the cross-plane direction is nearly a 1,000 times weaker, limited by van der Waals interactions with the environment (for graphene) [4] or between graphene sheets (for graphite) [1] , [2] . Recent studies have suggested that the thermal conductivity of graphene is altered when in contact with a substrate through the interaction between vibrational modes (phonons) of graphene and those of the substrate [5] , [6] , [7] , [8] . However, an understanding of heat-flow properties in nanometre-scale samples of graphene (or any other two-dimensional (2D) materials) is currently lacking. By comparison, most graphene studies have focused on its electrical properties when confined to scales on the order of the carrier mean free path (mfp) [9] , [10] , [11] , [12] , [13] , [14] . For example, these studies have found that ‘short’ devices exhibit near-ballistic behaviour [9] and Fabry–Perot wave interference [12] , whereas ‘narrow’ nanoribbons display a steep reduction of charge-carrier mobility [11] , [13] . Previous studies do exist for heat flow in three-dimensional (3D) structures, such as nanowires and nanoscale films. For instance, ballistic heat flow was observed in suspended GaAs bridges [15] and silicon nitride membranes [16] at low temperatures, of the order 1 K. Conversely, suppression of thermal conductivity due to strong edge-scattering effects was noted in narrow and rough silicon nanowires [17] , [18] , up to room temperature. Yet, such effects have not been studied in 2D materials like graphene, and ballistic heat conduction has not been previously observed near room temperature in any material. In this work we find that the thermal properties of graphene can be tuned in nanoscale devices comparable in size to the intrinsic phonon mfp. (By ‘intrinsic’ thermal conductivity or phonon mfp, we refer to that in large samples without edge effects, typically limited by phonon–phonon scattering in suspended graphene [3] and by substrate scattering in supported graphene [6] ; here λ ≈100 nm at room temperature, as we will show.) We find that the thermal conductance of ‘short’ quarter-micron graphene devices reaches up to 35% of theoretical ballistic upper limits [19] . However, the thermal conductivity of ‘narrow’ graphene nanoribbons (GNRs) is greatly reduced compared with that of ‘large’ graphene samples. Importantly, we uncover that nanoengineering the GNR dimensions and edges is responsible for altering the effective phonon mfp, shifting heat flow from quasi-ballistic to diffusive regimes. These findings are highly relevant for all nanoscale graphene devices and interconnects, also suggesting new avenues to manipulate thermal transport in 2D and quasi-one-dimensional systems. 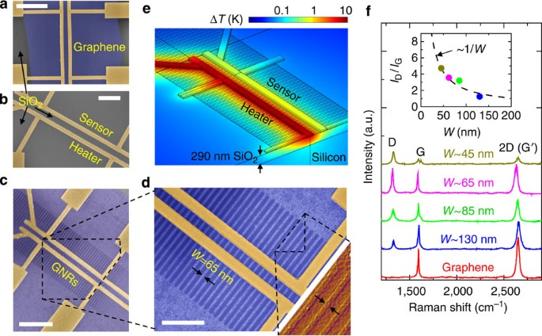Figure 1: Measurement of heat flow in graphene ribbons. (a) Scanning electron microscopy image of parallel heater and sensor metal lines with ~260 nm separation, on top of graphene sample (colourized for emphasis). A thin SiO2layer under the metal lines provides electrical insulation and thermal contact with the graphene beneath (see Methods andSupplementary Note S1). (b) Similar sample after graphene etch, serving as control measurement for heat flow through contacts and SiO2/Si underlayers. (c) Heater and sensor lines across array of graphene nanoribbons (GNRs). (d) Magnified portion of array with GNR widths ~65 nm; inset shows atomic force microscopy image of GNRs. Scale bars ofa–d, 2, 1, 2 and 1 μm, respectively. (e) 3D simulation of experimental structure, showing temperature distribution with current applied through heater line. (f) Raman spectra of unpatterned graphene sample (bottom curve) and GNRs (upper curves, offset for clarity). Inset shows scaling of Raman D to G peak area versus GNR width, consistent with the enhanced role of edge disorder in narrower GNRs14,21,35. Test structures and measurements Figure 1 illustrates several of our experimental test structures, showing graphene and GNR arrays supported on a SiO 2 /Si substrate (see Methods and Supplementary Note S1 ). Long, parallel metal lines serve as heater and thermometer sensors [5] , [20] , electrically insulated from the graphene by a thin SiO 2 layer. We perform heat-flow measurements from 20 to 300 K on unpatterned graphene ( Fig. 1a ), control samples with the graphene etched off ( Fig. 1b ) and arrays of GNR widths W ≈130, 85, 65 and 45 nm ( Fig. 1c and Supplementary Fig. S2 ). Figure 1f shows the Raman spectra of representative samples, with no discernible D peak (no defects) in unpatterned graphene [4] and a D/G peak ratio of GNRs consistent with the presence of edge disorder [14] , [21] . Figure 1: Measurement of heat flow in graphene ribbons. ( a ) Scanning electron microscopy image of parallel heater and sensor metal lines with ~260 nm separation, on top of graphene sample (colourized for emphasis). A thin SiO 2 layer under the metal lines provides electrical insulation and thermal contact with the graphene beneath (see Methods and Supplementary Note S1 ). ( b ) Similar sample after graphene etch, serving as control measurement for heat flow through contacts and SiO 2 /Si underlayers. ( c ) Heater and sensor lines across array of graphene nanoribbons (GNRs). ( d ) Magnified portion of array with GNR widths ~65 nm; inset shows atomic force microscopy image of GNRs. Scale bars of a – d , 2, 1, 2 and 1 μm, respectively. ( e ) 3D simulation of experimental structure, showing temperature distribution with current applied through heater line. ( f ) Raman spectra of unpatterned graphene sample (bottom curve) and GNRs (upper curves, offset for clarity). Inset shows scaling of Raman D to G peak area versus GNR width, consistent with the enhanced role of edge disorder in narrower GNRs [14] , [21] , [35] . Full size image The measurement proceeds as follows. We pass a heating current through one metal line, which sets up a temperature gradient across the sample, and we monitor changes in electrical resistance of the opposite electrode (see Methods and Supplementary Note S2 ). Both electrode resistances are calibrated over the full temperature range for each sample, allowing us to convert measured changes of resistance into changes of sensor temperature Δ T S , as a function of heater power P H ( Supplementary Fig. S5 ). We also perform measurements after removing the exposed graphene with an oxygen plasma etch ( Fig. 1b ). This allows us to obtain the thermal properties of the parallel heat-flow path through the contacts, supporting SiO 2 and substrate ( Supplementary Figs S4 and S8 ). As a check on our method, we find the thermal conductivity of our SiO 2 layer in excellent agreement with well-known data from the literature ( Supplementary Note S4 and Supplementary Fig. S8 ) over the full temperature range. As a result of this exercise, we were also able to fit the thermal resistance of the SiO 2 –Si interface ( Supplementary Fig. S8c and Supplementary Eq. S1 ), generating one of the few available data sets on this quantity, to our knowledge. To extract the thermal properties of our samples, we use 3D simulations of the structures with dimensions obtained from measurements by scanning electron microscopy and atomic force microscopy, as shown in Fig. 1d and Supplementary Fig. S7 . The model matches the measured and simulated Δ T S and P H , fitting the thermal conductance G between the heater and the thermometer. The 3D simulations automatically include all known contact-resistance effects, including those of the graphene–SiO 2 and SiO 2 –metal interfaces, matched against data from the literature and our control experiments ( Supplementary Note S3 ). To provide some simple estimates, the contact thermal resistance (per electrode width) is R C ≈0.7 m. KW −1 , the ‘wide’ unpatterned graphene thermal resistance is R G ≈2.5 m. KW −1 and that of the GNR arrays is in the range R GNR ≈4–32 m. KW −1 (from widest to narrowest). The graphene is not patterned under the electrodes; thus, the contact resistance remains the same for all samples. The 3D simulations also account for heat spreading through the underlying SiO 2 , and our error bars include various uncertainties in all parameters ( Supplementary Note S6 ). 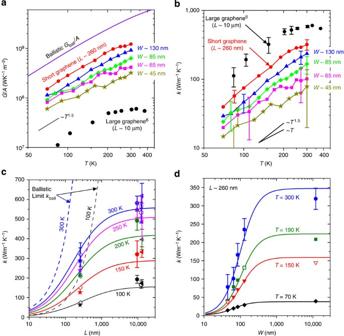Figure 2: Thermal conduction scaling in GNRs. (a) Thermal conductance per cross-sectional area (G/A) versus temperature for our GNRs (L≈260 nm,Was listed, seeFig. 3c), a ‘short’ unpatterned sample (L≈260 nm,W≈12 μm, seeFig. 3b) and a ‘large’ sample from Seolet al.6(L≈10 μm,W≈2.4 μm, seeFig. 3a). The short but wide graphene sample attains up to ~35% of the theoretical ballistic heat-flow limit22,23,24(also seeSupplementary Fig. S9). (b) Thermal conductivity for the same samples as ina(also seeSupplementary Fig. S10). (c) Thermal conductivity reduction with length for ‘wide’ samples (Wλ), compared with the ballistic limit (kball=GballL/A) at several temperatures. Symbols are data for our ‘short’ unpatterned graphene samples (Figs 1aand3b), and ‘large’ samples of Seolet al.6(Fig. 3a). Solid lines are model from equation 1. (d) Thermal conductivity reduction with width for GNRs, all withL≈260 nm (Figs 1c,dand3c). Solid symbols are experimental data fromb, open symbols are interpolations for the listed temperature. Lines are fitted model from equation 2, revealing a scaling as ~W1.80.3in the edge-limited regime. The thermal conductivity of plasma-etched GNRs in this work appears slightly lower than that estimated for GNRs from unzipped nanotubes13at a given width, consistent with a stronger effect of edge disorder35. Also seeSupplementary Fig. S11. Figure 2a displays in-plane thermal conductance per area ( G / A ) for our GNRs, for one of our unpatterned ‘short but wide’ samples ( L ≈260 nm, W ≈12 μm), and for the ‘large’ sample ( L ≈10 μm) of Seol et al . [6] Here A is the cross-sectional area of heat flow, A = WH , where W is the width and H =0.335 nm is the thickness of the graphene samples. At the same time Fig. 3 displays schematics of the size effects and the three transport regimes expected, corresponding to the samples measured in Fig. 2 . Figure 2a also shows the theoretical ballistic thermal conductance of graphene [22] , [23] , [24] , G ball / A , calculated with the approach listed in Supplementary Note S9 . By comparison, our ‘short’ sample (schematic in Fig. 3b ) has a thermal conductance ~35% of G ball / A at 200 K and ~30% at room temperature, indicating a regime of quasi-ballistic phonon transport (other similar samples are shown in Supplementary Fig. S9d ). In contrast, the ‘large’ sample from Seol et al . [6] (schematic in Fig. 3a ) has a conductance per cross-sectional area <2% of the ballistic limit, being in the diffusive transport regime as expected ( W , L ≫ λ ). Figure 2: Thermal conduction scaling in GNRs. ( a ) Thermal conductance per cross-sectional area ( G / A ) versus temperature for our GNRs ( L ≈260 nm, W as listed, see Fig. 3c ), a ‘short’ unpatterned sample ( L ≈260 nm, W ≈12 μm, see Fig. 3b ) and a ‘large’ sample from Seol et al . [6] ( L ≈10 μm, W ≈2.4 μm, see Fig. 3a ). The short but wide graphene sample attains up to ~35% of the theoretical ballistic heat-flow limit [22] , [23] , [24] (also see Supplementary Fig. S9 ). ( b ) Thermal conductivity for the same samples as in a (also see Supplementary Fig. S10 ). ( c ) Thermal conductivity reduction with length for ‘wide’ samples ( W λ ), compared with the ballistic limit ( k ball = G ball L / A ) at several temperatures. Symbols are data for our ‘short’ unpatterned graphene samples ( Figs 1a and 3b ), and ‘large’ samples of Seol et al . [6] ( Fig. 3a ). Solid lines are model from equation 1. ( d ) Thermal conductivity reduction with width for GNRs, all with L ≈260 nm ( Figs 1c,d and 3c ). Solid symbols are experimental data from b , open symbols are interpolations for the listed temperature. Lines are fitted model from equation 2, revealing a scaling as ~ W 1.8 0.3 in the edge-limited regime. The thermal conductivity of plasma-etched GNRs in this work appears slightly lower than that estimated for GNRs from unzipped nanotubes [13] at a given width, consistent with a stronger effect of edge disorder [35] . Also see Supplementary Fig. S11 . 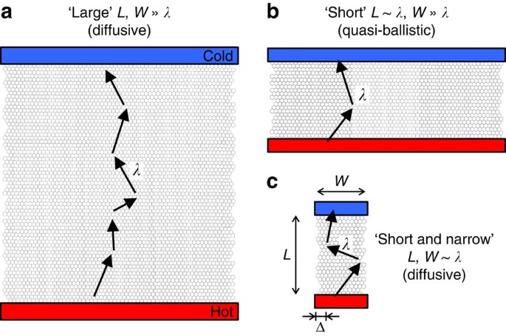Figure 3: Schematic of size effects and different heat-flow regimes. (a) Diffusive heat transport in ‘large’ samples with dimensions much greater than the intrinsic phonon mfp (L,Wλ). This regime corresponds to the samples measured in both substrate-supported6and -suspended graphene2,3studies to date. (b) Quasi-ballistic heat flow in ‘short but wide’ samples (L~λandWλ). This regime corresponds to our geometry shown inFig. 1a, withL≈260 nm andW≈12 μm. (c) Return to a diffusive heat transport regime as the sample width is narrowed down, and phonon scattering with edge roughness (of r.m.s. Δ) begins to dominate. This regime corresponds to our arrays of GNRs fromFig. 1c–e(L≈260 nm andWvarying from 45 to 130 nm). A fourth regime (longL, narrowW) is not shown here, but it can be easily understood from the above. Full size image Figure 3: Schematic of size effects and different heat-flow regimes. ( a ) Diffusive heat transport in ‘large’ samples with dimensions much greater than the intrinsic phonon mfp ( L , W λ ). This regime corresponds to the samples measured in both substrate-supported [6] and -suspended graphene [2] , [3] studies to date. ( b ) Quasi-ballistic heat flow in ‘short but wide’ samples ( L ~ λ and W λ ). This regime corresponds to our geometry shown in Fig. 1a , with L ≈260 nm and W ≈12 μm. ( c ) Return to a diffusive heat transport regime as the sample width is narrowed down, and phonon scattering with edge roughness (of r.m.s. Δ) begins to dominate. This regime corresponds to our arrays of GNRs from Fig. 1c–e ( L ≈260 nm and W varying from 45 to 130 nm). A fourth regime (long L , narrow W ) is not shown here, but it can be easily understood from the above. Full size image Length dependence of thermal conductivity We recall that in the ballistic limit ( L λ ), the conductance, rather than the conductivity, approaches a constant at a given temperature [22] , [23] , [24] , G ball ( T ). Nevertheless, the thermal conductivity is the parameter typically used for calculating heat transport in practice, and for comparing different materials and systems. Thus, the well-known relationship k =( G / A ) L imposes the conductivity k to become a function of length in the ballistic regime and to decrease as L is reduced. This situation becomes evident when we plot the thermal conductivity in Fig. 2b , finding k ≈320 W m −1 K −1 for our ‘short’ and wide samples at room temperature (schematic Fig. 3b ), almost a factor of two lower than the large graphene [6] (schematic Fig. 3a ). We note that both unpatterned samples here and in Seol et al . [6] were supported by SiO 2 , showed no discernible defects in the Raman spectra and the measurements were repeated over three samples ( Supplementary Note S5 and Supplementary Fig. S9 ), with similar results obtained each time. The transition of 2D thermal conductivity from diffusive to ballistic can be captured through simple models [25] , similar to the apparent mobility reduction during quasi-ballistic charge transport observed in short-channel transistors [26] , [27] : The first equality is a ‘three-colour’ model with p the phonon mode (longitudinal acoustic; transverse; flexural), G p,ball calculated using the appropriate dispersion [19] and ∑ k p,diff = k diff the diffusive thermal conductivity (~600 W m −1 K −1 at 300 K) [6] . A simpler ‘gray’ approximation can also be obtained by dropping the p index, k ( L )≈[ A /( LG ball )+1/ k diff ] −1 , where G ball / A ≈4.2 × 10 9 W K −1 m −2 at room temperature [19] (see Supplementary Note S9 ). The second expression in equation 1 is a Landauer-like model [25] , [28] , with π /2 accounting for angle averaging [29] in 2D to obtain the phonon backscattering mfp. For convenience, we note that the ballistic thermal conductance of graphene can be approximated analytically as G ball / A ≈[1/(4.4 × 10 5 T 1.68 )+1/(1.2 × 10 10 )] −1 W K −1 m −2 over the temperature range 1–1,000 K, as a fit to full numerical calculations ( Supplementary Fig. S16 ). We compare the simple models in equation 1 with the experiments in Fig. 2c and find good agreement over a wide temperature range. The comparison also yields our first estimate of the intrinsic phonon mfp in SiO 2 -supported graphene, λ ≈(2/ π ) k diff /( G ball / A )≈90 nm at 300 K and 115 nm at 150 K. (The same argument estimates an intrinsic phonon mfp λ ≈300–600 nm in freely suspended graphene at 300 K, if a thermal conductivity 2,000–4,000 W m −1 K −1 is used [1] , [2] , [3] .) This phonon mfp is the key length scale which determines when the thermal conductivity of a sample becomes a function of its dimensions, in other words when L and W become comparable to λ . On the basis of Fig. 2c , we note that quasi-ballistic heat-flow effects should become non-negligible in all SiO 2 -supported graphene devices shorter than ~1 μm. Width dependence of thermal conductivity We now turn to the width dependence of heat flow in narrow GNRs. Our experimental data in Fig. 2b show a clear decrease of thermal conductivity as the width W is reduced to a size regime comparable to the intrinsic phonon mfp. For instance, at room temperature k ≈230, 170, 100 and 80 W m −1 K −1 for GNRs of W ≈130, 85, 65 and 45 nm, respectively, and same L ≈260 nm. To understand this trend, we consider k limited by phonon scattering with edge disorder [30] , [31] through a simple empirical model with a functional form suggested by previous work on rough nanowires [32] , [33] and GNR mobility [34] : Here Δ is the root-mean-square (r.m.s.) edge roughness ( Fig. 3c ) and k ( L ) is given by equation 1. The solid lines in Fig. 2d show good agreement with our GNR data ( L ≈260 nm) using Δ=0.6 nm and a best-fit exponent n =1.8±0.3. The parameter c =0.04 W m −1 K −1 can be used to fit the room-temperature data set and additional fitting discussion is provided in the Supplementary Note S9 . (Note that we cannot assign an overly great physical meaning to the parameter c , because the empirical model can only fit Δ n / c , not Δ or c independently). The simple model appears to be a good approximation in a regime with Δ W , where the data presented here were fitted. However, it is likely that this simple functional dependence would change in a situation with extreme edge roughness [18] , where the roughness correlation length (which cannot be directly quantified here) could also have an important role. Nevertheless, the nearly W -squared dependence of thermal conductivity in narrow GNRs with edge roughness is consistent with previous findings for rough nanowires [32] , [33] , and also similar to that suggested by theoretical studies of GNR electron mobility [34] . The precise scaling with Δ is ostensibly more complex [30] , [31] than can be captured in a simple model, as it depends on details of the phonon dispersion, the phonon wave vector and indirectly on temperature. However, the Δ estimated from the simple model presented above is similar to that from extensive numerical simulations below, and to that measured by transmission electron microscopy on GNRs prepared under similar conditions [35] . Thus, the simple expressions given above can be taken as a practical model for heat flow in substrate-supported GNRs with edge roughness (Δ W ) over a wide range of dimensions, corresponding to all size regimes in Fig. 3 . We first revisit the effects of measurement contacts and how they relate to the interpretation of sample length in the quasi-ballistic heat-flow regime. As in studies of quasi-ballistic electrical transport [26] , [27] , we defined the ‘channel length’ L as the inside edge-to-edge distance between the heater and thermometer electrodes ( Fig. 3c ). Simple ballistic theory assumes contacts with an infinite number of modes and instant thermalization of phonons at the edges of the contacts. The former is well approximated here by electrodes two hundred times thicker than the graphene sheet; however, phonons may travel some distance below the contacts before equilibrating. The classical, continuum analogue of this aspect is represented by the thermal transfer length ( L T ) of heat flow from the graphene into the contacts [3] , [36] , which is automatically taken into account in our 3D simulations ( Fig. 1e ). However, a subcontinuum perspective [37] reveals that graphene phonons only thermally equilibrate after travelling one mfp below the contacts. Previous measurements of oxide-encased graphene [5] had estimated a thermal conductivity k enc =50–100 W m −1 K −1 , which suggests a phonon mfp λ enc =(2 k enc / π )/( G ball / A )≈8–15 nm under the contacts. This adds at most 12% to our assumption of edge-to-edge sample length (here L ≈260 nm), a small uncertainty which is comparable to the sample-to-sample variation from fabrication, and to the size of the symbols in Fig. 2c . (The relatively low thermal conductivity of encased monolayer graphene [5] is due to scattering with the SiO 2 sandwich, although some graphene damage from the SiO 2 evaporation [38] on top is also possible.) To gain deeper insight into our experimental results, we employ a numerical solution of the Boltzmann transport equation (BTE) with a complete phonon dispersion [31] , [39] . Our approach is similar to previous work [6] , [40] , but accounting for quasi-ballistic phonon propagation and edge disorder scattering in short and narrow GNRs, respectively (see Methods and Supplementary Notes S7 and S8 ). 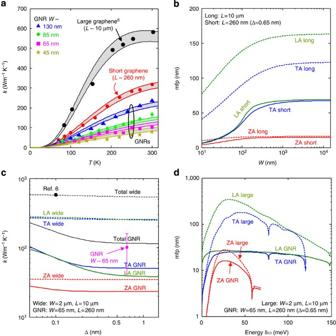Figure 4: Insights from numerical simulations. (a) Comparison of Boltzmann transport model (lines) with experimental data (symbols, same asFig. 2b, but here on linear scale). (b) Computed scaling of phonon mfp versus width, for two sample lengths as listed. Longitudinal acoustic (LA) and transverse (TA) phonons with long intrinsic mfp are subject to stronger size effects from edge scattering than flexural (ZA) modes, which are primarily limited by substrate scattering. (c) Estimated contribution of modes to thermal conductivity versus edge roughness Δ for a wide sample and a narrow GNR. Similar toW, changes in Δ also more strongly affect LA and TA modes, until substrate scattering begins to dominate. (d) Phonon mfp versus energy (frequency) for a large sample and a narrow GNR. Low-frequency modes are strongly affected by substrate scattering, such that effects of edge roughness are most evident forħω>15 meV. Panelsb–dare all at room temperature. Also seeSupplementary Figs S13 and S15. Figure 4a finds good agreement of thermal conductivity between our measurements and the BTE model across all samples and temperatures. We obtained the best fit for GNRs of width 130 and 85 nm with r.m.s. edge roughness Δ=0.25 and 0.3 nm, where the gray bands in Fig. 4a correspond to ±5% variation around these values. For GNRs of widths 65 and 45 nm, the gray bands correspond to edge roughness ranges Δ=0.35–0.5 and 0.5–1 nm, respectively. We note that unlike the empirical model of equation 2, the best-fit BTE simulations do not use a unique value of edge roughness Δ. This could indicate some natural sample-to-sample variation in edge roughness from the fabrication conditions, but it could also be due to certain edge-scattering physics (such as edge-roughness correlation [18] and phonon localization [41] ), which are not yet captured by the BTE model. Figure 4: Insights from numerical simulations. ( a ) Comparison of Boltzmann transport model (lines) with experimental data (symbols, same as Fig. 2b , but here on linear scale). ( b ) Computed scaling of phonon mfp versus width, for two sample lengths as listed. Longitudinal acoustic (LA) and transverse (TA) phonons with long intrinsic mfp are subject to stronger size effects from edge scattering than flexural (ZA) modes, which are primarily limited by substrate scattering. ( c ) Estimated contribution of modes to thermal conductivity versus edge roughness Δ for a wide sample and a narrow GNR. Similar to W , changes in Δ also more strongly affect LA and TA modes, until substrate scattering begins to dominate. ( d ) Phonon mfp versus energy (frequency) for a large sample and a narrow GNR. Low-frequency modes are strongly affected by substrate scattering, such that effects of edge roughness are most evident for ħω >15 meV. Panels b – d are all at room temperature. Also see Supplementary Figs S13 and S15 . Full size image Figure 4b examines the scaling of mfps by phonon mode, finding they are strongly reduced as the GNR width decreases below ~200 nm, similar to the thermal conductivity in Fig. 2d . The mfp for each phonon mode is calculated as an average over the entire frequency spectrum, weighted by the frequency-dependent heat capacity and group velocity ( Supplementary Eq. S19 ). We note that longitudinal acoustic (LA) and transverse (TA) modes, which have larger intrinsic mfps, are more strongly affected by the GNR edge disorder. On the other hand, flexural acoustic modes (ZA) are predominantly limited by substrate scattering and consequently suffer less from edge disorder, consistently with recent findings from molecular dynamics simulations [7] , [8] . Increasing edge disorder reduces phonon mfps ( Supplementary Fig. S15d ), and the thermal conductivity is expected to scale as shown in Fig. 4c . In the BTE model, the edge-roughness scattering is captured using a momentum-dependent specularity parameter ( Supplementary Eq. S11 ), meaning that small wavelength (large momentum q ) phonons are more strongly affected by line edge roughness. However, as Δ increases the specularity parameter saturates, marking a transition to fully diffuse edge scattering, and also to a regime where substrate scattering begins to dominate long-wavelength phonons in substrate-supported samples. This transition cannot be captured by the simplified Δ n dependence in the empirical model of equation 2. To further illustrate such distinctions, Fig. 4d displays the energy (frequency ω ) dependence of phonon mfps for a ‘small’ GNR and a ‘large’ SiO 2 -supported graphene sample (corresponding to Fig. 3c and 3a , respectively). Low-frequency substrate scattering (proportional to ~1/ ω 2 ) dominates the large sample [6] , [7] , whereas scattering with edge disorder affects phonons with wavelengths comparable to, or smaller than, the roughness Δ (see Supplementary Note S7 ). Therefore, larger Δ can affect more long-wavelength (low energy) phonons, but only up to Δ~1 nm, where the effect of the substrate begins to dominate in the long-wavelength region (also seen in Fig. 4c ). Such a separation of frequency ranges affected by substrate and edge scattering could provide an interesting opportunity to tune both the total value and the spectral components of thermal transport in GNRs, by controlling the substrate and edge roughness independently. Finally, it is instructive to examine some similarities and differences between our findings here versus previous results regarding size effects on charge-carrier mobility in GNRs with dimensions comparable to the phonon or electron mfp. The edge-limited thermal conductivity begins to fall off in GNRs narrower than ~200 nm ( Fig. 2d ), or twice the intrinsic phonon mfp. A similar trend was noted for the electrical mobility in GNRs [11] , but with a fall off at widths narrower than ~40 nm ( Supplementary Fig. S11 ). These observations are consistent with the intrinsic electron mfp being several times shorter [13] , [42] than the phonon mfp in SiO 2 -supported graphene, that is, ~20 nm for the electron mfp versus nearly ~100 nm for the phonon mfp at room temperature. Thus, edge disorder affects thermal transport more strongly than charge transport in GNRs of an intermediate width (40< W <200 nm), an effect that could be used to manipulate charge and heat flow independently in such nanostructures. In conclusion, we have investigated heat flow in SiO 2 -supported graphene samples of dimensions comparable to the phonon mfp. Short devices ( L ~ λ , corresponding to Fig. 3b schematic) have thermal conductance much higher than that previously found in micron-sized samples, reaching 35% of the ballistic limit at 200 K and 30% (~1.2 GW K −1 m −2 ) at room temperature. However, narrow ribbons ( W ~ λ , corresponding to Fig. 3c schematic) show decreased thermal conductivity due to phonon scattering with edge disorder. Thus, the usual meaning of thermal conductivity must be carefully interpreted when it becomes a function of sample dimensions. The results also suggest powerful means to tune heat flow in 2D nanostructures through the effects of sample width, length, substrate interaction and edge disorder. Sample fabrication Graphene monolayers were deposited on SiO 2 /Si (~290 nm/0.5 mm) substrates by mechanical exfoliation from natural graphite. Graphene thickness and GNR edge disorder were evaluated with Raman spectroscopy [4] , [21] , [35] . Samples were annealed in Ar/H 2 at 400 °C for 40 min. Electron (e)-beam lithography was used to pattern the heater and thermometer electrodes as long, parallel, ~200-nm-wide lines with current and voltage probes, with a separation of L ≈260 nm ( Fig. 1 ). Electrodes were deposited by successive evaporation of SiO 2 (20 nm) for electrical insulation and Ti/Au (30/20 nm) for temperature sensing. Additional e-beam lithography and oxygen plasma etching were performed when needed, to define GNR arrays with pitch ~150 nm and varying widths. Electrical and thermal measurements The heater electrode is slowly ramped up (<0.2 mHz) to 1.5 mA. We measured the resistance change of the sensor electrode through a lock-in technique with a frequency of 2,147 Hz and r.m.s. current of 1 μA (carefully verified to avoid additional heating). All electrical measurements were performed in a four-probe configuration, inside a Physical Property Measurement System (Quantum Design). Numerical simulation We obtain the thermal conductivity by solving the Boltzmann transport equation in the relaxation time approximation, including scattering at the rough GNR edges [31] . The simulation uses the phonon dispersion of an isolated graphene sheet, which is a good approximation for SiO 2 -supported graphene within the phonon frequencies that contribute most to transport [8] , and at typical graphene–SiO 2 interaction strengths [7] . (However, we note that artificially increasing the graphene–SiO 2 coupling, for example, by applying pressure [43] , could lead to modifications of the phonon dispersion and hybridized graphene–SiO 2 modes [7] .) We assume a graphene monolayer thickness H =0.335 nm and a concentration of 1% 13 C isotope point defects [2] , [6] . The interaction with the SiO 2 substrate is modelled through perturbations to the scattering Hamiltonian [6] at small patches where the graphene is in contact with the SiO 2 , with nominal patch radius a =8.75 nm. Anharmonic three-phonon interactions of both normal and umklapp type are included in the relaxation time (see Supplementary Note S7 ). An equivalent 2D ballistic scattering rate [25] , [29] ~2 v x / L is used in the numerical solution (x is the heat flow direction along graphene) to account for transport in short GNRs. How to cite this article: Bae, M.-H. et al . Ballistic to diffusive crossover of heat flow in graphene ribbons. Nat. Commun. 4:1734 doi: 10.1038/ncomms2755 (2013).